Dynamic evolution of venom proteins in squamate reptiles Phylogenetic analyses of toxin gene families have revolutionised our understanding of the origin and evolution of reptile venoms, leading to the current hypothesis that venom evolved once in squamate reptiles. However, because of a lack of homologous squamate non-toxin sequences, these conclusions rely on the implicit assumption that recruitments of protein families into venom are both rare and irreversible. Here we use sequences of homologous non-toxin proteins from two snake species to test these assumptions. Phylogenetic and ancestral-state analyses revealed frequent nesting of 'physiological' proteins within venom toxin clades, suggesting early ancestral recruitment into venom followed by reverse recruitment of toxins back to physiological roles. These results provide evidence that protein recruitment into venoms from physiological functions is not a one-way process, but dynamic, with reversal of function and/or co-expression of toxins in different tissues. This requires a major reassessment of our previous understanding of how animal venoms evolve. Squamate venoms are complex mixtures of protein and peptide components (commonly referred to as toxins) that act to kill or immobilise prey, and may possibly aid in digestion. The origin of the venom apparatus of squamates has been the subject of considerable recent research interest. The homology of the venom apparatus across the advanced snakes (Caenophidia) is robustly supported by anatomical evidence [1] , [2] , [3] , [4] , as well as comparative embryology and developmental genetics [5] . A recent addition to the body of evidence supporting the single early evolution of venom in snakes has been the use of protein amino acid or DNA gene sequences from toxins, and their homologues among non-venom body proteins [6] , [7] . Venom toxins belong to multiple multi-locus gene families, evolving according to the birth and death model [8] , and first acquired their role within venom following recruitment from protein families fulfilling ordinary physiological functions [9] . Mapping the gene tree of these protein families onto the corresponding organismal tree allows the reconstruction of the history of the recruitment of the toxin into the venomous arsenal of the animals. This approach provided additional support for the single early evolution of venom in the Caenophidia [7] . Among lizards, only the genus Heloderma (family Helodermatidae) was considered to be venomous until very recently. As the venom apparatus of Heloderma is confined to the lower jaw, whereas that of snakes is restricted to the upper jaw, the two systems had always been assumed to be non-homologous. However, this assumption was challenged by Fry et al . [10] , who identified toxin-secreting glands in the lower jaws of additional lizards of the families Varanidae and Anguidae, and in both upper and lower jaws of representatives of the Iguania. As these three groups, together with the Helodermatidae and Serpentes (snakes), form a monophyletic group, Fry et al . [10] postulated a single early origin (SEO) of venom at the base of that clade, termed the Toxicofera (see Supplementary Fig. S1 for a phylogeny of the Toxicoferan reptiles). However, in the absence of strong morphological or developmental evidence of homology between the upper jaw glands of iguanian lizards and snakes, the key piece of evidence for the single origin of venom rested with toxin gene phylogenies, which showed the monophyly of lizard and snake toxin genes to the exclusion of non-venom homologues, and in some cases the lack of reciprocal monophyly of snake and lizard toxins [10] . The major problem with the interpretation of these gene phylogenies is the lack of comparable sequences of non-venom homologues from within the Toxicofera. In the absence of available genomic sequences, non-toxin homologues of the venom toxins in these studies were derived from a variety of other vertebrate taxa, most commonly mammals or birds [7] , [9] , [10] , [11] , [12] . This is potentially problematic, because failure to sample non-toxin homologues from the focal clade can lead to gene trees that falsely depict the toxin genes as monophyletic, leading to the erroneous conclusion that they are the result of a single recruitment event ( Fig. 1a,b ) The rigorous testing of toxin monophyly in any protein family therefore requires the inclusion of non-toxin homologues from within the focal clade ( Fig. 1c ). 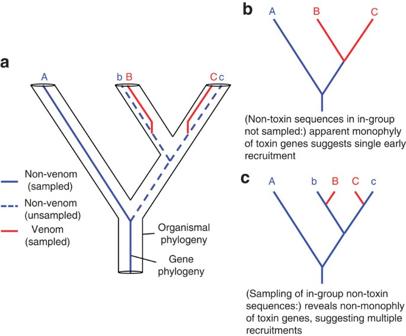Figure 1: Potential effect of sampling non-venom proteins. Diagram showing the potential effect of sampling non-venom proteins from in-group taxa on the interpretation of toxin recruitment. (a) Actual gene family evolution within organismal phylogeny; (b) effect of non-inclusion of non-toxin sequences: gene tree suggests single early recruitment of toxin genes into venom; (c) sampling of non-toxin sequences from in-group reveals non-monophyly of toxins, suggesting multiple independent recruitment events. Figure 1: Potential effect of sampling non-venom proteins. Diagram showing the potential effect of sampling non-venom proteins from in-group taxa on the interpretation of toxin recruitment. ( a ) Actual gene family evolution within organismal phylogeny; ( b ) effect of non-inclusion of non-toxin sequences: gene tree suggests single early recruitment of toxin genes into venom; ( c ) sampling of non-toxin sequences from in-group reveals non-monophyly of toxins, suggesting multiple independent recruitment events. Full size image Two additional key assumptions that have remained untested due to the lack of non-toxin homologues from previous studies are that changes of role from physiological function into venom are rare in protein family evolution, and that there is no 'reverse recruitment' of toxin proteins back into a physiological role. Consequently, the current narrative of venom evolution rests on two key assumptions that have remained untested, again largely due to the lack of available in-group, non-toxin sequences. Recently, Toxicoferan non-toxin sequences have become available, thanks to transcriptomic studies involving multiple organs of one Caenophidian ( Thamnophis elegans [13] ), and heart and liver tissue from a basal snake ( Python bivittatus , as P. molurus bivittatus [14] ). Here, we use these new sequences of physiological proteins sourced from non-venom gland tissues to rigorously test the hypothesis of an early recruitment of nine toxin families into the venom arsenal of squamate reptiles. Evidence of toxin monophyly following the inclusion of sampled non-toxin gene homologues will provide strong support for the SEO hypothesis proposed by Fry et al . [10] In contrast, evidence of toxin non-monophyly (that is, non-toxins nesting within toxin clades) would indicate that either multiple origins of venom have occurred in the squamate reptiles or that the recruitment of proteins into the venom gland may not be a one-way process, but also involve reverse recruitment of toxins into non-venom functions outside the venom gland. To explicitly test these hypotheses, we utilised rigorous phylogenetic analyses alongside ancestral character state reconstructions to investigate the origin of venom, and the nature and frequency of recruitments into and from a toxin function in squamate venom protein families. Toxin and non-toxin sequences BLAST sequence searches of the non-toxin transcriptome libraries revealed hits to T. elegans contiguous sequences (contigs) for eight toxin families (crotamine, cobra venom factor (CVF), cystatin, hyaluronidase, kallikrein, lectin, nerve growth factor (NGF) and veficolin) and four to P. bivittatus contigs (CVF, hyaluronidase, kallikrein and NGF). The natriuretic toxin family was retained for analysis despite an absence of hits, because of the existence of toxin-like sequences previously isolated from the brain tissue of a snake species ( Bothrops jararaca ). Sequence alignments for each toxin family (containing Toxicoferan toxins, Toxicoferan non-toxins and outside-group gene homologues) resulted in the following DNA and amino acid data sets: crotamine – 17 sequences, 345 DNA positions, 115 amino acid positions; CVF – 32 sequences, 1619 DNA positions, 540 amino acid positions; cystatin – 40 sequences, 510 DNA positions, 170 amino acid positions; hyaluronidase – 24 sequences, 1411 DNA positions, 470 amino acid positions; kallikrein – 65 sequences, 1320 DNA positions, 441 amino acid positions; lectin – 27 sequences, 543 DNA positions, 181 amino acid positions; natriuretic – 48 sequences, 1122 DNA positions, 374 amino acid positions; NGF – 29 sequences, 1092 DNA positions, 383 amino acid positions; veficolin – 18 sequences, 1065 DNA positions, 358 amino acid positions. Interpretations of the differences in Bayes factors generated by unpartitioned data sets and those partitioned by codon position strongly advocated the use of partitioned models of sequence evolution for phylogenetic analyses ( Supplementary Table S1 ). Models of sequence evolution assigned by MrModelTest [15] and ModelGenerator [16] that were utilised in phylogenetic analyses are displayed in Supplementary Table S2 . Tracer [17] revealed that the point of convergence (burnin) for Bayesian analyses had occurred before the first 1.5×10 6 generations for all parameters, but we conservatively discarded these generations and calculated the consensus trees from the remaining 75% of the posterior distribution. All parameters of the Tracer analyses had effective sample sizes above 200 and in the vast majority of cases by a large margin. Phylogenetic analyses The results of phylogenetic analyses of each gene family by Bayesian inference [18] and maximum likelihood [19] of DNA and amino acid datasets are displayed in Figs 2 , 3 , 4 , 5 and Supplementary Figs S2–S6 . Table 1 summarises the tree topologies observed in these figures, including where evidence of Toxicoferan or snake toxin monophyly was observed. Out of the nine putatively basal toxin families analysed, none exhibited a Toxicoferan toxin clade that is monophyletic to the exclusion of all non-toxin homologues – in all gene families, physiological proteins sampled from non-venom gland tissues were found nested among toxin sequences. This was the result of sequences isolated from T. elegans in eight gene families (crotamine, CVF, cystatin, hyaluronidase, kallikrein, lectin, NGF, veficolin), sequences isolated from P. bivittatus in three gene families (CVF, kallikrein, NGF) and sequences isolated from other snakes in two gene families (CVF, natriuretic). 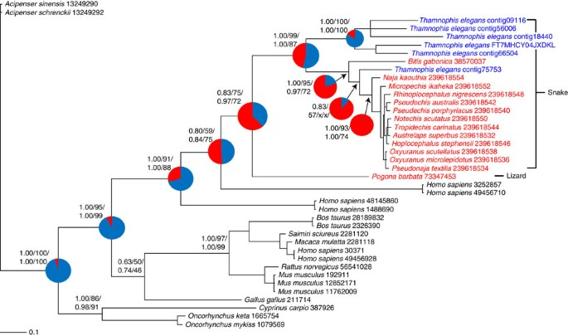Figure 2: Bayesian DNA gene tree of the cystatin toxin family. Multiple support values are given at key nodes in the following order: Bayesian DNA, maximum likelihood (ML) DNA, Bayesian amino acid (aa), ML aa; x indicates no support for the node in that analysis. Tips of the tree coloured in red indicate Toxicoferan sequences sourced from the venom gland and those coloured in blue indicate the ones sourced from non-venom gland tissues ('physiological' non-toxins). Pie charts represent the bpp of ancestral state reconstructions at that node: red=venom, blue=non-venom. The numbered codes for each sequence presented in the genetree represent GenBank GI accession numbers. Using Bayes factors to compare the observed (unconstrained) tree topologies with those in which Toxicoferan toxins were constrained to be monophyletic resulted in the rejection of toxin monophyly in all nine gene families ( Table 2 ). In addition, only two gene families (crotamine and veficolin) exhibited evidence of snake toxin monophyly ( Table 1 and Supplementary Figs S2 and S6 ). In all other toxin families, non-toxin sequences (that is, T. elegans or \ P. bivittatus physiological proteins expressed in non-venom gland tissues) were observed nested within snake toxin clades ( Figs 2 , 3 , 4 , 5 and Supplementary Figs S3–S5 ). Utilising Bayes factors to compare the observed tree topologies with those constrained to produce monophyly of snake toxins resulted in the rejection of snake toxin monophyly in five of the nine toxin families ( Table 2 ). In addition to crotamine and veficolin, we could not reject the possibility of snake toxin monophyly in the cystatin and hyaluronidase gene families. Figure 2: Bayesian DNA gene tree of the cystatin toxin family. Multiple support values are given at key nodes in the following order: Bayesian DNA, maximum likelihood (ML) DNA, Bayesian amino acid (aa), ML aa; x indicates no support for the node in that analysis. Tips of the tree coloured in red indicate Toxicoferan sequences sourced from the venom gland and those coloured in blue indicate the ones sourced from non-venom gland tissues ('physiological' non-toxins). Pie charts represent the bpp of ancestral state reconstructions at that node: red=venom, blue=non-venom. The numbered codes for each sequence presented in the genetree represent GenBank GI accession numbers. 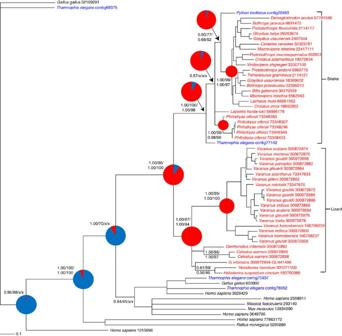Figure 3: Bayesian DNA gene tree of the kallikrein toxin family. Multiple support values are given at key nodes in the following order: Bayesian DNA, ML DNA, Bayesian aa, ML aa; x indicates no support for the node in that analysis. Tips of the tree coloured in red indicate Toxicoferan sequences sourced from the venom gland and those coloured in blue indicate the ones sourced from non-venom gland tissues ('physiological' non-toxins). Pie charts represent the bpp of ancestral state reconstructions at that node: red=venom, blue=non-venom. The numbered codes for each sequence presented in the genetree represent GenBank GI accession numbers. Full size image Figure 3: Bayesian DNA gene tree of the kallikrein toxin family. Multiple support values are given at key nodes in the following order: Bayesian DNA, ML DNA, Bayesian aa, ML aa; x indicates no support for the node in that analysis. Tips of the tree coloured in red indicate Toxicoferan sequences sourced from the venom gland and those coloured in blue indicate the ones sourced from non-venom gland tissues ('physiological' non-toxins). Pie charts represent the bpp of ancestral state reconstructions at that node: red=venom, blue=non-venom. The numbered codes for each sequence presented in the genetree represent GenBank GI accession numbers. 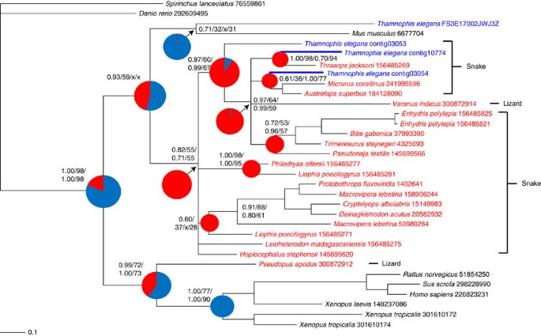Figure 4: Bayesian DNA gene tree of the lectin toxin family. Multiple support values are given at key nodes in the following order: Bayesian DNA, ML DNA, Bayesian aa, ML aa; x indicates no support for the node in that analysis. Tips of the tree coloured in red indicate Toxicoferan sequences sourced from the venom gland and those coloured in blue indicate the ones sourced from non-venom gland tissues ('physiological' non-toxins). Pie charts represent the bpp of ancestral state reconstructions at that node: red=venom, blue=non-venom. Positive selection detected on non-toxin branches is indicated by bold blue branches (T. eleganscontig10774,P=0.002 andT. eleganscontig03054,P=0.031 – likelihood ratio test with three degrees of freedom). The numbered codes for each sequence presented in the genetree represent GenBank GI accession numbers. Full size image Figure 4: Bayesian DNA gene tree of the lectin toxin family. Multiple support values are given at key nodes in the following order: Bayesian DNA, ML DNA, Bayesian aa, ML aa; x indicates no support for the node in that analysis. Tips of the tree coloured in red indicate Toxicoferan sequences sourced from the venom gland and those coloured in blue indicate the ones sourced from non-venom gland tissues ('physiological' non-toxins). Pie charts represent the bpp of ancestral state reconstructions at that node: red=venom, blue=non-venom. Positive selection detected on non-toxin branches is indicated by bold blue branches ( T. elegans contig10774, P =0.002 and T. elegans contig03054, P =0.031 – likelihood ratio test with three degrees of freedom). The numbered codes for each sequence presented in the genetree represent GenBank GI accession numbers. 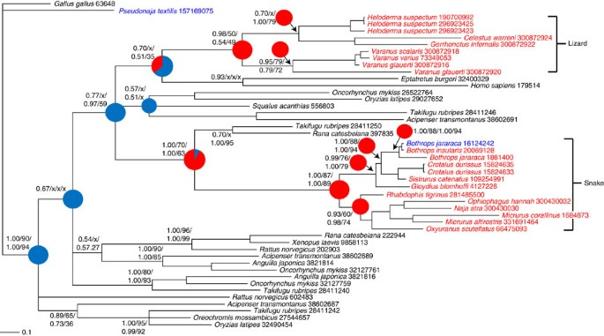Figure 5: Bayesian DNA gene tree of the natriuretic toxin family. Multiple support values are given at key nodes in the following order: Bayesian DNA, ML DNA, Bayesian aa, ML aa; x indicates no support for the node in that analysis. Tips of the tree coloured in red indicate Toxicoferan sequences sourced from the venom gland and those coloured in blue indicate the ones sourced from non-venom gland tissues ('physiological' non-toxins). Pie charts represent the bpp of ancestral state reconstructions at that node: red=venom, blue=non-venom. The numbered codes for each sequence presented in the genetree represent GenBank GI accession numbers. Full size image Figure 5: Bayesian DNA gene tree of the natriuretic toxin family. Multiple support values are given at key nodes in the following order: Bayesian DNA, ML DNA, Bayesian aa, ML aa; x indicates no support for the node in that analysis. Tips of the tree coloured in red indicate Toxicoferan sequences sourced from the venom gland and those coloured in blue indicate the ones sourced from non-venom gland tissues ('physiological' non-toxins). Pie charts represent the bpp of ancestral state reconstructions at that node: red=venom, blue=non-venom. The numbered codes for each sequence presented in the genetree represent GenBank GI accession numbers. Full size image Table 1 Results of phylogenetic analyses and ancestral node reconstructions of nine putatively basal Toxicoferan toxin families. Full size table Table 2 Comparison of alternative phylogenetic hypotheses of nine toxin families using Bayes factors. Full size table Ancestral state reconstruction To differentiate between the hypotheses of multiple recruitments into venom and single recruitment followed by reversals, the ancestral state reconstruction of venom as a character was undertaken for each key node present in the gene trees [20] . The Bayesian posterior probability of ancestral phylogenetic nodes representing venom toxins are displayed as percentage pie charts mapped onto the gene trees ( Figs 2 , 3 , 4 , 5 and Supplementary Figs S2–S6 ). Table 1 summarises the support that ancestral reconstruction analyses of each gene family provided for the SEO of venom in squamate reptiles, and independent origins of venom in snakes and lizards. Support for the SEO hypothesis [10] was observed in six of the nine gene families, although substantial support (Bayesian posterior probabilities (bpp) >0.95) was only observed in one of these (the lectin gene family). Nonetheless, kallikrein (0.90), NGF (0.85) and, to a lesser extent, crotamine (0.74) and hyaluronidase (0.73) provide additional, albeit weaker, support for this hypothesis. Among the remaining three gene families, analyses of CVF and veficolin failed to distinguish between the two hypotheses with any level of support, whereas the natriuretic gene family exhibited substantial support for the independent recruitment of these toxins in snakes and lizards ( Table 1 and Fig. 5 ). Ancestral reconstruction analyses also indicated that the placement of non-toxin sequences within toxin clades is not the result of multiple independent recruitments of toxins into the venom gland. In eight of the nine gene families analysed, they supported venom as the character state at nodes found at the base of clades containing both toxin and non-toxin sequences ( Table 1 ; Figs 2 , 3 , 4 , 5 ; Supplementary Figs S2–S5 ). Four were strongly supported (bpp >0.95 – kallikrein, lectin, natriuretic, NGF), whereas three provided reasonable support (bpp=0.78–0.89) for the hypothesis that toxin genes are capable of 'reverse recruitment' back into physiological tissues from the venom gland. The remaining toxin family (crotamine) exhibited weak support for this hypothesis (bpp=0.65). Detection of adaptive molecular evolution Tests of positive selection were undertaken for each non-toxin branch nested within toxins clades present in the gene trees ( Figs 2 , 3 , 4 , 5 ; Supplementary Figs S2–S6 ) to assess whether adaptive molecular evolution above background levels could be detected. Significant ( P ≤0.05) evidence of positive selection was observed in two independent branches in the lectin gene tree ( P =0.002 and 0.031 – likelihood ratio (LR) test with three degrees of freedom; Fig. 4 and Supplementary Table S3 ), providing strong evidence that these non-toxin proteins have evolved by adaptive evolution. In contrast, the remaining toxin families analysed revealed little evidence of positive selection above background levels acting on non-toxin branches present in the gene trees ( Supplementary Table S3 ). The results of the inclusion of a substantial body of Toxicoferan physiological protein sequences (empirically sampled from non-venom gland tissues) in the analysis of toxin gene family phylogenies require a reassessment of the origin of squamate venom systems, and of the relationship between the function and site of expression of venom proteins and their close non-toxin homologues. Instead of rare recruitment events from a physiological function into a venom function, our data suggest a much more dynamic relationship between 'internal' functions in the physiology of the producer animal and 'external' functions as venoms injected into other organisms. The results of our phylogenetic analyses revealed evidence of non-toxin sequences nesting among toxins in each gene family sampled, thereby providing strong evidence for the non-monophyly of Toxicoferan toxins ( Table 1 ; Figs 2 , 3 , 4 , 5 ; Supplementary Figs S2–S6 ). This is further supported by evidence that tree topologies constrained to show the monophyly of Toxicoferan toxins are strongly rejected when compared with unconstrained tree topologies ( Table 2 ). If we were to interpret these surprising results based on the current assumption that the recruitment of proteins into a toxin function is both rare and a one-way process (that is, with no reverse recruitment of toxins back to a physiological role), the results of our phylogenetic analyses would strongly refute the key prediction of the 'SEO' hypothesis for the Toxicoferan venom delivery system [10] , namely that the venom toxins in each protein family should form a monophyletic group to the exclusion of physiological (non-venom) proteins. However, our results also revealed that only two of the nine toxin families (crotamine and veficolin) contained a strongly supported monophyletic clade of snake toxins ( Table 1 ), although the monophyly of snake toxins was also not rejected in the cystatin and hyaluronidase gene trees ( Table 2 ). As the single origin of venom in advanced snakes is strongly supported by multiple independent sources of evidence [2] , [4] , [5] , this suggests that the non-monophyly of their toxins may instead be due to multiple, independent recruitment events or as the result of reverse recruitment. Logically, those same phenomena, rather than multiple independent origins of venom, may also be responsible for the non-monophyly of Toxicoferan toxins. To test this hypothesis and distinguish between multiple independent recruitments into venom and reverse recruitments back to a physiological role, we reconstructed the evolutionary history of character states at ancestral nodes within the gene trees. Six of the nine toxin families analysed exhibited support for the SEO of venom in the Toxicofera ( Table 1 ), indicating that the presence of non-toxin sequences nested within toxin clades in each of these trees results from one or several reversals rather than multiple independent recruitment events. In contrast, the SEO hypothesis was only rejected for the natriuretic toxin family, where we found strong support for independent recruitment events in the lizards and snakes. Moreover, the ancestral state reconstruction in eight of the nine toxin families provided support (four substantially – bpp >0.95) for the hypothesis that the reverse recruitment of venom toxins back into physiological tissues, or co-expression of toxins in different tissues, is responsible for the observed absence of toxin monophyly ( Table 1 ). Our data thus support the novel hypothesis that reverse recruitment and/or co-expression of toxin-encoding genes may be common in squamates. Distinguishing whether 'reverse recruitment' (where a duplicated locus is recruited back into a non-venom function) or protein co-expression (where the same locus is expressed in multiple tissue types) is responsible for the observed nesting of non-toxins within clades of toxin genes is problematic in the absence of gene sequences isolated from both venom and non-venom gland tissues from the same species. However, the nesting of P. bivitattus non-toxin sequences within toxin clades in the kallikrein and NGF toxin families ( Fig. 3 ; Supplementary Fig. S5 ) is important, because this species does not have a venom gland, following its secondary loss over evolutionary time; this clearly excludes the possibility of simple co-expression. Notably, in the kallikrein toxin family, the phylogenetic position of the P. bivitattus sequence is well supported (bpp=0.90), with strong support also observed for venom as the ancestral condition at the node preceding this branch (bpp=0.97; Fig. 3 ). The placement of the P. bivitattus NGF sequence within the Toxicoferan toxin clade was also strongly supported (bpp=1.00), although support for the single origin of venom was lower (bpp=0.85; Supplementary Fig. S5 ). Nonetheless, the combination of these results, where non-venom sequences sampled from a non-venomous species are found nested within toxin clades, provide strong support for the hypothesis that the reverse recruitment of proteins from the ancestral venom gland back to physiological tissues has occurred in at least some toxin families. In addition, neofunctionalisation of a reverse-recruited protein from 'toxin' back to 'non-toxin' can be predicted to result in positive selection acting on the gene in question (although this is not a prerequisite): evidence of positive selection acting upon those branches in the gene tree would therefore support the reverse-recruitment hypothesis. Consequently, we utilised positive selection tests to investigate whether adaptive evolution could be detected in any of the non-toxin branches present within each of the gene trees. Notably, despite the limitations of the approach in this specific instance (in particular the fact that the analysis only detects evidence of excess selection in the branches of interest over background levels – the latter of which are likely to be high, as most toxin genes evolve by positive selection [21] , [22] , [23] ), we detected significant evidence of adaptive evolution acting on two independent non-toxin branches present in the lectin gene tree ( Fig. 4 ; Supplementary Table S3 ). This evidence of excess positive selection over an already high background level is consistent with the predictions of neofunctionalisation of the proteins involved. Alongside the results of our phylogenetic analyses and ancestral state reconstructions of venom evolution, this provides further support for our hypothesis that, in at least some toxin families, venom proteins have been reverse recruited for physiological expression in non-venom gland tissues. Detecting evidence of reverse recruitment is perhaps not that surprising, as venom toxins are typically originally recruited into the venom gland by gene duplication of a physiological gene [9] . Here we propose that the same process may be responsible for some instances of reverse recruitment, with a gene expressed in the venom gland being duplicated (which occurs frequently in a number of toxin families [21] , [22] , [23] , [24] , [25] , [26] ) and undergoing adaptive evolution to neofunctionalise the encoded protein for physiological expression ( Fig. 6 ). However, it remains undetermined whether these 'reverse-recruited' proteins are physiologically expressed in the same tissue types that the proteins were originally recruited from into the venom gland [9] , and what the functional activities of the 'reverse-recruited' proteins are and how they compare with the ancestral physiological gene homologues or the toxins from which they originate. Future studies experimentally verifying differences in the site of expression and the functional activities of 'reverse-recruited' proteins, their ancestral physiological homologues and the toxins from which they originate will be particularly revealing. 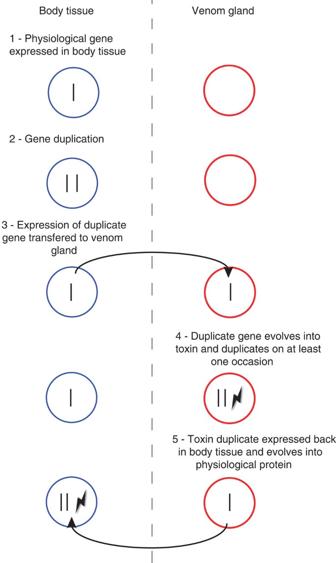Figure 6: Gene processes and the evolutionary history of Toxicoferan toxins. Schematic of the gene process likely involved in the evolutionary history of some Toxicoferan toxins and their non-toxin homologues. Blue circles=body tissue; red circles=venom gland; vertical line=gene; arrows=gene recruitment; lightning=positive selection. Figure 6: Gene processes and the evolutionary history of Toxicoferan toxins. Schematic of the gene process likely involved in the evolutionary history of some Toxicoferan toxins and their non-toxin homologues. Blue circles=body tissue; red circles=venom gland; vertical line=gene; arrows=gene recruitment; lightning=positive selection. Full size image Aside from multiple branches in the lectin gene tree, the remaining toxin families revealed little evidence of positive selection acting on non-venom branches ( Supplementary Table S3 ), complicating remaining interpretations of non-toxins nested within toxin clades in the gene trees. Although inherent technical limitations (see above) may have prevented the detection of additional non-toxin branches exhibiting evidence of positive election, we cannot rule out the possibility that the phylogenetic placement of some non-toxin genes is the result of co-expression of a gene in both the venom gland and other tissues. Interestingly, a natriuretic peptide isolated from the brain of Bothrops jararaca (GenBank GI accession: 16124242 ) [27] exhibited 97% sequence similarity to a venom protein isolated from the closely related species B. insularis (GenBank GI accession: 20069128 ; Fig. 5 ). This raises the intriguing possibility that, in addition to reverse recruitment, co-expression of some venom genes may also be occurring, although we cannot exclude the possibility that some venom proteins may only require minor changes (not requiring positive selection) to revert back from a role in venom to an 'internal' physiological function. Nevertheless, evidence of high sequence similarity between non-toxin and toxin homologues in some gene families and evidence of positive selection acting on non-toxins in others suggest that perhaps a combination of these processes are responsible for the complex and dynamic evolutionary histories observed here. Previous studies of venom evolution have relied on the implicit assumption that recruitment events into a toxin role are both rare and irreversible events. Our results for the lectin and natriuretic toxin families suggest that protein recruitment into venom may be more frequent than previously thought: at least two recruitment events have occurred in the lectins, once at the base of the Toxicofera and another in the lizard Pseudopus ( Ophisaurus ) apodus ( Fig. 4 ), and independent recruitments of natriuretic peptides have occurred in the snakes and lizards ( Fig. 5 ). In addition, if reverse recruitment back to a physiological function indeed explains the gene trees obtained, then such reverse recruitment events from venom back to physiological tissues may also be fairly common, with non-toxin body proteins often observed as non-monophyletic in the gene trees (for example, Figs 2 , 3 , 4 ; Supplementary Figs S3, S5, S6 ) and evidence of positive selection acting on independent branches in the lectin toxin family ( Supplementary Table S3 ). However, we stress that the sequencing of Toxicoferan non-toxin proteins remains in its infancy, and that additional transcriptomic or genomic studies may require a revision of this interpretation, particularly in reference to the inferred number of 'recruitment events' occurring between venom and non-venom gland tissues and in terms of assessing the relative importance of reverse recruitment and co-expression. The discovery that the recruitment of expressed genes between 'internal' (body tissue) physiological functions and 'external' venom systems appears to be a dynamic and reversible process ( Fig. 6 ) has important biological implications beyond the origin of reptilian venoms. For example, our data suggest that some physiological proteins present in members of the venomous reptiles may be a great source for investigation as new targets for drug discovery. A number of venom toxins have been successfully exploited for medical purposes as a result of their potent biological activities [28] . Toxin isoforms that have reverted back to a physiological function may share these functional potencies as a result of their common origin, yet have presumably subsequently evolved to be functionally non-toxic for expression in a vertebrate physiological system. Consequently, such proteins may provide model targets for future pharmacological investigation, as well as providing an excellent system for the investigation of the changes involved in the acquisition and loss of toxicity in proteins. In conclusion, our results reveal an unexpectedly dynamic mode of evolution occurring in some reptilian toxin families, including the first evidence that venom toxin derivatives are physiologically expressed for a 'non-toxic' role and, in some cases, their possible co-expression in multiple tissues. These insights require a reconsideration of how biochemical weapon systems, such as venom, evolve in the natural world, and provide a basis for further exploration of the evolutionary dynamics of neofunctionalisation in the evolution of protein families. Toxin and non-toxin sequences Body tissue homologues of Toxicoferan venom (toxin) gene families were identified by nucleotide BLAST searches of assembled contigs available from T. elegans (a multiple organ archive) and P. bivittatus (heart and liver) transcriptomic libraries [13] , [14] . The T. elegans data set were searched using the Bronikowski Lab Data Server ( http://eco.bcb.iastate.edu/ ), whereas P. bivittatus contigs were downloaded from the snake genomics webpage ( http://www.snakegenomics.org/ ) and formatted into a BLAST-able database. Both databases were interrogated using representative venom sequences utilised by Fry et al [10] , [11] , [12] , [29] . Sequence searches were undertaken for 12 toxin families identified as basal to the Toxicofera (AVIT, cystatin, cysteine-rich secretory protein, CVF, crotamine, hyaluronidase, kallikrein, lectin, natriuretic peptides, NGF, veficolin and vespryn) [10] , [11] , [12] . Contigs exhibiting a BLAST e -value cut-off of 1e−05 were retained. BLAST hits to natriuretic, cysteine-rich secretory protein and vespryn were not found in either transcriptomic database. Additional non-venom gland sequences previously isolated from snake physiological tissues were also incorporated into the data sets ( Supplementary Table S4 ). Contig hits were incorporated into DNA data sets of toxin (derived from members of the Toxicofera) and non-toxin (sampled from outside groups – that is, non-reptilian species) sequences used in the analyses of Fry et al [10] , [11] , [12] , [29] . All sequences were obtained from GenBank – GI accession numbers are displayed in the resulting gene trees ( Figs 2 , 3 , 4 , 5 ; Supplementary Figs S2–S6 ). Because of the paucity of toxin sequences available for CVF, cystatin and natriuretic at the time of original analysis [10] , we incorporated additional, recently published sequences for these protein families to rigorously test our hypotheses. The AVIT toxin family was excluded from further analyses owing to a very small sample size and complete absence of DNA sequences from snakes. DNA data sets were trimmed to the open-reading frame in MEGA5 (ref. 30 ), with identical sequences and those containing truncations or frameshifts (as the result of insertions or deletions) excluded. Each DNA data set was tested for evidence of recombination in the recombination detection programme RDP3 v3.44 (ref. 31 ). Standard parameters were utilised for the RDP, GENECONV and Bootscan methods using a P -value cut-off of 0.05 and sequences exhibiting a positive signal excluded from further analysis ( Supplementary Table S5 ). Subsequently, each data set was aligned by MUSCLE [32] and the alignments checked manually before phylogenetic analysis. Amino acid data sets were constructed by the translation of DNA sequences and realignment with MUSCLE [32] . Phylogenetic analyses DNA and amino acid gene trees for each toxin family were generated using Bayesian inference and maximum likelihood methodologies. Considering complex models of sequence evolution have been demonstrated to extract additional phylogenetic signal from data [33] , [34] , we subjected the DNA data sets to codon analysis in MrModelTest v2.3 (ref. 15 ) and the amino acid data sets in ModelGenerator v0.85 (ref. 16 ). The model favoured under the Akaike Information Criterion [35] was selected for incorporation into Bayesian inference analyses. Bayesian analyses were undertaken using a Markov Chain Monte Carlo algorithm in MrBayes v3.1 (ref. 18 ) on the freely available bioinformatic platform Bioportal ( www.bioportal.uio.no [36] ). Each data set was run in duplicate using four chains simultaneously (three heated and one cold) for 5×10 6 generations, sampling every 500th cycle from the chain and using default settings in regards to priors. Tracer v1.4 (ref. 17 ) was used to estimate effective sample sizes for all parameters and to construct plots of ln( L ) against generation to verify the point of convergence (burnin); trees generated before the completion of burnin were discarded. To avoid potential overparameterisation as a result of implementing multiple codon models of sequence evolution [37] , [38] , we compared Bayes factors generated by Bayesian inference analysis of codon partitioned and unpartitioned (utilising a single model of sequence evolution selected by MrModelTest [15] and, second, utilising a mixed model) data sets in Tracer [17] , [39] . Bayes factors are defined as the likelihood of data under a particular model after parameter estimation from two competing hypotheses – comparisons of Bayes factors can be interpreted as the success of each hypothesis at predicting the data [40] , [41] . The marginal log-likelihoods for each Bayesian analysis were retrieved, Bayes factors of codon partitioned and unpartitioned data sets were calculated in Tracer [17] and the results interpreted based on previously described guidelines [40] . For maximum likelihood, we used RAxML-VI-HPC2 v7.2.7 on teragrid at the CIPRES Science Gateway ( www.phylo.org ) [19] , [42] . For each data set, analyses were conducted using 100 alternative runs with nonparametric bootstrap analysis (500 replicates) used to provide branch support values for the most likely tree. DNA data sets utilised the Generalised time-reversible (GTR) gamma model, whereas amino acid analyses incorporated the CAT model and the protein substitution matrix selected by ModelGenerator analysis. Other parameters were maintained at default settings. Testing alternative hypotheses The significance of constraining gene trees that did not originally support the monophyly of Toxicoferan toxin and snake toxin sequences was explored using Bayes factors to quantify the support of alternative hypotheses [39] . Here, the null hypotheses were the optimal gene trees resulting from unconstrained DNA Bayesian analyses. These trees were compared with those representing the alternative hypothesis – trees produced in an identical manner, with the exception of tree topologies constrained to produce either a monophyly of Toxicoferan toxins or snake toxins. The resulting Bayes factors were compared and interpreted as outlined above. Ancestral state reconstructions Bayesian ancestral state reconstructions were undertaken in SIMMAP v1.5.2 using stochastic mutational mapping under the ancestral states criterion to predict the posterior probability of the state of a character at each ancestral node in the tree [20] , [43] . This method accounts for phylogenetic uncertainty in the gene tree by sampling tree topologies, branch lengths, model parameters and character histories. The posterior probability that an ancestral node has a venom character state was assessed by allocating a single character (venom=1 and non-venom=0) to the tips on the tree, based on the tissue location each sequence was sourced from. The ancestral reconstruction of venom as a character at each node was assessed using 1,000 rooted post-burnin trees sampled from the posterior distribution of the Bayesian analyses for each DNA data set. We used a low rate prior which incorporated a mean of 1 and a s.d. of 5 of the prior distribution; the number of samples and stochastic draws from this prior distribution was set at 50 (refs 43 , 44 ). Detection of adaptive molecular evolution We modified the 'test 2' branch-site method of Zhang et al . [45] to test the hypothesis that toxin-related sequences that have been putatively recruited to a non-toxin role will exhibit evidence for positive Darwinian change. Specifically, we classified background branches a priori as toxin and foreground branches as non-toxin. Under the null hypothesis, there are two classes of sites corresponding to purifying natural selection (0<ω 0 <1) and neutral ( ω 1 =1) which apply homogeneously across the tree. Under the alternate hypothesis, there are two additional classes of sites that were both adaptively evolving ( ω 2 >1) on the non-toxin edge, but on the toxin edges were subjected to either purifying selection or neutral evolution. Thus, the alternate hypothesis has three additional parameters: ω 2 and two additional site-class probability terms. We evaluated whether the data were adequately explained by the null hypothesis using a standard LR test. In this instance, the LR statistic is asymptotically χ 2 -distributed with three degrees of freedom. The major modification over the original form of Zhang et al . [45] is that we employ the conditional nucleotide form of the codon rate matrix [46] . We used the conditional nucleotide form variant that includes terms from the nucleotide general time reversible model, as it was demonstrated as the form most robust to changes in sequence composition [46] . This model assumes codons evolve independently and that the substitution processes is stationary and reversible. For each toxin family, a separate hypothesis test was performed for each putative non-toxin sequence. In the cases where there were multiple non-toxin edges, only the one non-toxin edge was included in the data at a time. Data used for the tests for positive selection were a subset of those used for phylogenetic reconstruction. To ensure a minimum amount of information conferred by sequences, only those with at least 60 unambiguously sequenced bases where included. To reduce computation time and improve the accuracy of parameter estimates, we pruned the phylogenetic trees in two ways. For sequences that had close relatives in the data set, as indicated by very short (for example, 0) branch lengths, single representatives with the most sequenced bases were chosen. Where possible, we eliminated branches with excessive divergence (branch lengths>1), as these branches are more prone to saturation of synonymous substitutions. Inclusion of such branches in the background will potentially cause underestimation of background ω and thus overestimation of foreground ω [47] , [48] , [49] . All tests of selection were implemented using PyCogent version 1.5.1 (ref. 50 ). For each alignment, the DNA tree derived from Bayesian inference phylogenetic analysis was used. Those trees were also used to identify putative target branches for changed positive selection by virtue of their recruitment to a non-venom function. We employed the conventional treatment for modelling aligned columns with gaps, treating them as missing data. Codon frequencies were included as free parameters in the model and estimated from the data. For the adaptively evolving site classes, we set an upper bound of 100 for ω . Maximum-likelihood estimates from the null model were used as initial values for the alternate model. Maximisation of models was done using a combination of simulated annealing and Powell numerical optimizers [50] . Initial optimisation was performed using simulated annealing followed by Powell, with maximum of five restarts and an exit condition tolerance of 1e−8. All of the models fit here satisfied this exit condition. We verified the consistency of the results by repeating the model-fitting process and comparing parameter estimates and likelihoods. Sequential Bonferroni corrections [51] were applied independently to each data set to account for any type-I error – significance of the test required the P- value of each branch to fall beneath the significance threshold calculated for each data set. All source codes, alignments and trees used for this analysis are available on request from the authors. How to cite this article: Casewell, N.R. et al . Dynamic evolution of venom proteins in squamate reptiles. Nat. Commun. 3:1066 doi: 10.1038/ncomms2065 (2012).